Atmospheric phosphorus deposition may cause lakes to revert from phosphorus limitation back to nitrogen limitation Recent findings indicate that increased atmospheric deposition of nitrogen of human origin has caused changes in the pattern of ecological nutrient limitation in lakes in the northern hemisphere. An increase in the nitrogen to phosphorus ratio, and hence a shift from pristine nitrogen limitation to human-induced phosphorus limitation of phytoplankton growth, seems to have been driven by deposition of atmospheric nitrogen. These findings challenge the classical paradigm of lake phytoplankton productivity being naturally limited by phosphorus availability. However, atmospheric phosphorus deposition may also be highly relevant. Here we show how dissolved inorganic nitrogen concentration has decreased in the Pyrenean lake district over recent decades, despite there being an increase in deposition of atmospheric nitrogen. This is related to an increased atmospheric phosphorus load in the lake water, as a result of higher atmospheric inputs. These changes are causing phytoplankton to revert from being phosphorus-limited to being nitrogen-limited. Humans have dramatically disturbed the earth's nitrogen (N) cycle [1] , [2] to the point that this alteration is considered one of the most serious threats to the global ecosystem [3] . Part of the excess N circulates through the atmosphere and is deposited with precipitation, reaching areas that would otherwise be free of direct human impact. Recent research has addressed the global impact of atmospherically deposited N as a nutrient [4] , [5] , [6] in lakes, showing that reactive N of human origin has caused an increase in the stoichiometric N/phosphorus (P) ratio, and hence a shift from N limitation to P limitation of phytoplankton growth. These findings challenge the classical paradigm of lake phytoplankton productivity being naturally limited by P availability, and support the notion put forward by Goldman [7] that P limitation of phytoplankton growth is a derived character induced by atmospheric N deposition. Supporting this hypothesis is the finding that there is a good correlation between dissolved inorganic N (DIN) deposition and lake water DIN concentration in a number of regions holding unproductive lakes in the northern hemisphere that receive increasing depositional loads [6] . However, deposition of atmospheric P may also be highly relevant. In contrast to what could be expected based on the aforementioned studies, DIN concentration has decreased in the Pyrenean lake district over recent decades, despite there being an increase in deposition of atmospheric N. Our measurements suggest that this observation is related to an increased atmospheric P load in the lake water, as a result of higher atmospheric inputs. These changes are causing the nutrient limitation status of phytoplankton to revert from being P-limited to being N-limited. Our data also indicate that increased P deposition responds to the meteorological conditions that facilitate the transport of dust from northern Africa and the Iberian Peninsula to the Pyrenees, thus revealing a mechanism by which changes in the movement of air masses interact with human emissions and eventually may change the nature of their impact on lake ecosystems. This biogeochemical effect probably influences the nutrient balance of lakes worldwide, with more pronounced effects in those locations receiving higher loads of atmospheric aerosols containing P of both natural and human origins [8] . Overall, our results demonstrate the need to consider the impact of global changes on ecosystems under an integrated perspective. An unexpected decreasing DIN trend in Pyrenean lakes Contrarily to what could be expected, data from several synoptic surveys in the Central Pyrenees spanning from 1987 to 2011 show a clear shift towards lower DIN concentration in lakes ( Fig. 1 ), while emissions of total N (NOx+NH 3 ) into the atmosphere in the area (which are the major source of deposited N) increased [9] ( Supplementary Fig. S1 ). 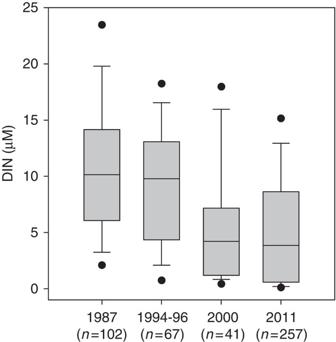Figure 1: Time trend of DIN in the Pyrenean lake district. Box plots showing the evolution of the distribution of DIN concentration in water from lakes in the central Pyrenees from 1987 to 2011. The box plots show medians (line within the box), 25th and 75th percentiles (sides of the box), 10th and 90th percentiles (error bars) and 5th and 95th percentiles (circles). Data are from four synoptic surveys carried out in the years indicated on the graph; the number of lakes included (n) is also indicated. The significance of the trend for the lake surveys data was tested by means of one-way analysis of variance (ANOVA) with trend contrast. DIN concentrations were first log transformed to normalize their distribution by years. Homogeneity of variances of the transformed variable was checked using Levene's statistic. One-way ANOVA test using the sampling year as a factor with four levels was conducted on the transformed data to test whether differences in means between years were different and to test whether there was a significant linear trend component across levels (in this case, sampling years). Differences between years were significant (F=31.792,P<0.001) and arranged according to a significant linear time trend (F=90.777,P<0.001). Figure 1: Time trend of DIN in the Pyrenean lake district. Box plots showing the evolution of the distribution of DIN concentration in water from lakes in the central Pyrenees from 1987 to 2011. The box plots show medians (line within the box), 25th and 75th percentiles (sides of the box), 10th and 90th percentiles (error bars) and 5th and 95th percentiles (circles). Data are from four synoptic surveys carried out in the years indicated on the graph; the number of lakes included ( n ) is also indicated. The significance of the trend for the lake surveys data was tested by means of one-way analysis of variance (ANOVA) with trend contrast. DIN concentrations were first log transformed to normalize their distribution by years. Homogeneity of variances of the transformed variable was checked using Levene's statistic. One-way ANOVA test using the sampling year as a factor with four levels was conducted on the transformed data to test whether differences in means between years were different and to test whether there was a significant linear trend component across levels (in this case, sampling years). Differences between years were significant (F=31.792, P <0.001) and arranged according to a significant linear time trend (F=90.777, P <0.001). Full size image The analysis of data from an intensively monitored catchment in the Central Pyrenees (Conangles catchment) provided insight into the processes involved in the DIN decrease in lakes. Lake Redon (formerly Lake Redó) lies in a Conangles subcatchment. Similarly to what we have observed for the whole lake district, we found that the DIN concentration in Lake Redon decreased while DIN deposition increased during the period 1998–2010 ( Fig. 2a,b ). The behaviour of the lake is also in contrast to the trend in Conangles creek, a stream which drains the Redon basin together with a much larger area without lakes. In spite of a relatively high year-to-year variability, the overall slope of the stream time-series followed that of deposition ( Fig. 2c ). This finding indicates that the terrestrial part of the catchment is not a N sink. Consequently, N exportation from terrestrial to aquatic systems is high and any decrease in lake-water DIN is attributable to causes within the lake. 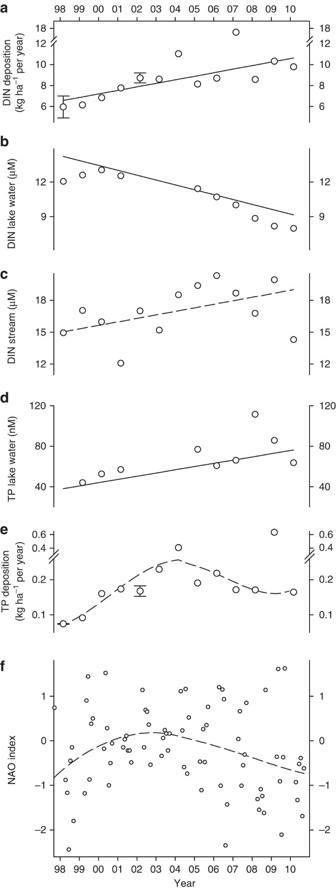Figure 2: Time trends of DIN and TP in the Conangles catchment. Time series of DIN in atmospheric deposition (a), Lake Redon (b) and Conangles creek (c); TP in Lake Redon (d) and in deposition (e); values for the monthly NAO index during the spring and summer (April–September) months (f). Chemical data (total deposition and average concentrations) are grouped by water years (that is, from 1 September–31 August). Note that the y axis break in (a) and (e). The error bars in (a) and (e) indicate the range of deposition measurements at two sampling stations. Straight lines (a–d) are the computed Kendall's overall trend lines, the solid ones indicating a high significance (P=0.004 for DIN deposition,P=0.001 for lake water DIN andP=0.029 for lake water TP) and the dashed line a nonsignificant trend (P=0.179 for the stream DIN). Curves (e,f) are local regression (LOESS) smoothing trend lines. The significance of linear trends was tested by mean of the nonparametric Mann–Kendall test, using the software provided by the US Geological Survey27. For nonlinear trends, trend lines were obtained as a smoothed LOESS curve (with sampling proportion=0.7, polynomial regression degree=2 and rejection of outliers). Figure 2: Time trends of DIN and TP in the Conangles catchment. Time series of DIN in atmospheric deposition ( a ), Lake Redon ( b ) and Conangles creek ( c ); TP in Lake Redon ( d ) and in deposition ( e ); values for the monthly NAO index during the spring and summer (April–September) months ( f ). Chemical data (total deposition and average concentrations) are grouped by water years (that is, from 1 September–31 August). Note that the y axis break in ( a ) and ( e ). The error bars in ( a ) and ( e ) indicate the range of deposition measurements at two sampling stations. Straight lines ( a – d ) are the computed Kendall's overall trend lines, the solid ones indicating a high significance ( P =0.004 for DIN deposition, P =0.001 for lake water DIN and P =0.029 for lake water TP) and the dashed line a nonsignificant trend ( P =0.179 for the stream DIN). Curves ( e , f ) are local regression (LOESS) smoothing trend lines. The significance of linear trends was tested by mean of the nonparametric Mann–Kendall test, using the software provided by the US Geological Survey [27] . For nonlinear trends, trend lines were obtained as a smoothed LOESS curve (with sampling proportion=0.7, polynomial regression degree=2 and rejection of outliers). Full size image Between 1998 and 2010, the total P (TP) concentration increased in Lake Redon ( Fig. 2d ), thereby indicating P fertilization, which may have stimulated N consumption. The deposition of TP also increased in this period ( Fig. 2e ), which is a possible cause of the trend observed in the lake. Changes in the recycling and internal load of P are alternative hypotheses to explain these observations; however, our monitoring of the general limnology of the lake does not support these alternative causes. In particular, changes in the duration of the ice cover or thermal stratification in the summer might be considered drivers of alterations of the P and N status of the lake. For instance, it could be hypothesized that longer hypolimnetic stagnation periods (either in winter or summer) lead to a greater release of P from sediments, although this would also be accompanied by a higher release of N, which was not found to be the case. It could also be speculated that longer ice-free periods involving a more extended period of phytoplankton growth caused the increased N consumption and consequent depletion observed. However, we did not detect a significant trend over the duration of the ice-free period (Kendall's τ =−0.164, P =0.533) or of the summer stratification ( τ =0.022, P =1.000) that could account for the trends observed in N and P ( Supplementary Figs S2 and S3 ). We therefore propose that increased external P input caused by atmospheric deposition is the most plausible explanation to account for our observations. Meteorological control on P deposition Overall, P deposition at the end of the study period roughly doubled that of the initial years. The concentration of P in the lake also doubled during the same period. However, the P deposition trend was not linear, showing a pronounced positive trend during 1998–2004 and some decrease afterwards. Dust transported from North Africa and also from the Iberian Peninsula appears to be the main source of atmospheric P deposited on Pyrenean watersheds. Previous studies have shown that there is a preferential flux of terrigenous elements accompanying precipitation of a southern origin [10] , [11] , [12] . A detailed study of the back trajectories of the air masses causing precipitation was conducted for 2004–2006 (ref. 12 ). During that period, only monthly precipitation samples containing >60% volume with a southern origin exhibited TP deposition values well above (up to >100 g P ha −1 ) a general background level (<10 g P ha −1 ), making up the bulk of yearly P deposition ( Fig. 3a ). Most high P deposition events occurred during spring and summer ( Fig. 3b ). Moulin et al . [13] found that there is a correlation ( r =0.66 and P =0.027, for data from 1982 to 1996) between atmospheric dust export from North Africa to the Mediterranean area and the climatic variability defined by the North Atlantic Oscillation (NAO). Consistent with this, for the spring and summer months from 1998 to 2010, the TP deposition followed, in general terms, the trend of the NAO index ( Fig. 2f ), thus confirming a certain meteorological control of P deposition over the Pyrenees. Months with a lower NAO index were more frequent at the beginning and end of the study period, thus reducing the probability of dust outbreaks towards the two ends. Intense dust outbreak episodes and subsequent deposition are, however, random. In addition, a single episode can contribute most of the yearly deposition, so outliers to the general trend can be expected. This was the case for the water year 2008–2009, when a single month (15 April 2009 to 11 May 2009) accounted for ~78% of the yearly P deposition (0.50 out of 0.63 kg ha −1 ), corresponding to a well-documented intense dust outbreak from 7 to 10 May 2009 (ref. 14 ). 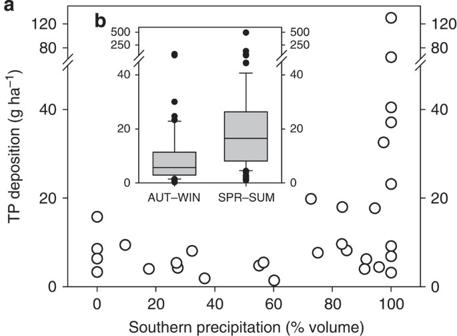Figure 3: Geographic origin and timing of TP deposition. TP deposition versus origin of the wet air masses causing precipitation from 2004 to 2006 (a) and seasonal TP deposition distributions during 1997–2010 (b). Note the y axis break in both graphs. In (a), circles represent 4-week bulk deposition samples from Lake Redon station. Each sample may be a composite of various events of distinct geographic origin occurring during the sampling period. The geographic assignment was done as follows. For each sample, the single events and their contribution to the final volume collected were determined using data from an on-site automatic weather station. A 72-h back trajectory was computed for each event using the HYSPLIT model28,29. The trajectories were then grouped on the basis of their origin, and the percentage of the volume corresponding to events assigned to groups with a southern origin was calculated for each sample12. Data in (b) are 4-week samples grouped in autumn–winter (AUT–WIN; October–March) and spring–summer (SPR–SUM; April–September) samples. The box plots show medians (line within the box), 25th and 75th percentiles (sides of the box), 10th and 90th percentiles (error bars) and all outliers (circles). Figure 3: Geographic origin and timing of TP deposition. TP deposition versus origin of the wet air masses causing precipitation from 2004 to 2006 ( a ) and seasonal TP deposition distributions during 1997–2010 ( b ). Note the y axis break in both graphs. In ( a ), circles represent 4-week bulk deposition samples from Lake Redon station. Each sample may be a composite of various events of distinct geographic origin occurring during the sampling period. The geographic assignment was done as follows. For each sample, the single events and their contribution to the final volume collected were determined using data from an on-site automatic weather station. A 72-h back trajectory was computed for each event using the HYSPLIT model [28] , [29] . The trajectories were then grouped on the basis of their origin, and the percentage of the volume corresponding to events assigned to groups with a southern origin was calculated for each sample [12] . Data in ( b ) are 4-week samples grouped in autumn–winter (AUT–WIN; October–March) and spring–summer (SPR–SUM; April–September) samples. The box plots show medians (line within the box), 25th and 75th percentiles (sides of the box), 10th and 90th percentiles (error bars) and all outliers (circles). Full size image Given the nonlinear trend in P deposition, the question arises as to how does it translate into a linear trend in the lake. Several arguments can be put forward. Atmospheric P deposition is highly episodic by nature, as mentioned above, and not all episodes influence the lake in the same way or with the same intensity. The effect of episodes depends on a variety of factors at a given moment, such as the hydrology and water circulation path through the lake, the productive stage of phytoplankton or the speciation of P that is supplied (in particular, the proportion of P bound to particles prone to rapid sedimentation), among other factors. A second consideration is that a large part of the atmospheric P is supplied through the catchment, which may act as a modulator. A final important deliberation is that the water renewal time of the lake is ~4 years, that is, any change observed in the lake chemistry integrates the previous 4-year history. All these points may explain the smoothed or delayed (or both) fluctuations in the atmospheric signal in the lake system, thereby resulting in a main response of a coincident doubling of P content, as mentioned above, but without necessarily reflecting all the nuances of the input signal. According to the theory of Bergström and Jannson [6] , lakes where phytoplankton is N-limited show a chlorophyll- a (Chla) to TP ratio that responds proportionally to increasing DIN, up to the point where they become P-limited. Beyond this point, the Chla/TP ratio remains constant with higher DIN. Therefore, the breakpoint between the two segments in a plot of DIN versus Chla/TP can be considered as a threshold between P and N limitation for phytoplankton. Pyrenean lakes lie on the threshold (98.4 μg N l −1 ≈7 μM DIN; Fig. 4 ) calculated from the data compiled in that study, with the inclusion of our own data (85 lakes) for this mountain range from the survey conducted in the year 2000. Consequently, being between P limitation and N limitation of phytoplankton, Pyrenean lakes are particularly sensitive to the ecological changes induced by varying depositional loads of N and P: the trend in lake-water DIN indicates that Lake Redon is now crossing the boundary; as for the whole central Pyrenean lake district, ~33% of lakes were below the threshold in 1987, whereas this percentage currently stands at ~70%. These observations potentially indicate that the phytoplankton from the lakes in the Pyrenees has shifted from being P-limited to N-limited. 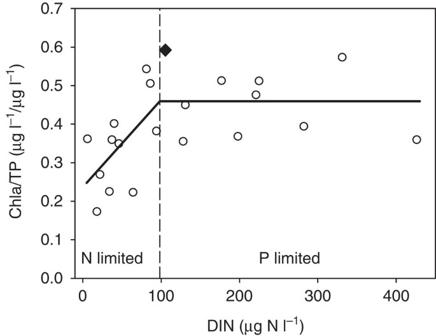Figure 4: The N- and P-limitation domains. The relationship between phytoplankton biomass (using Chla as a surrogate), TP and DIN are shown in this graph. The plotted data are regional averages of the ratio Chla/TP and DIN concentration for lakes in Europe and North America. This figure has been redrawn from the original source6, but using lake-water DIN instead of DIN deposition, and adding data from the survey performed in the Pyrenees in 2000 (diamond,n=85). The solid line is the segmented regression fit used to establish the optimum breakpoint (vertical dashed line) between the DIN-dependent and DIN-independent segments, calculated using SegReg software30. Figure 4: The N- and P-limitation domains. The relationship between phytoplankton biomass (using Chla as a surrogate), TP and DIN are shown in this graph. The plotted data are regional averages of the ratio Chla/TP and DIN concentration for lakes in Europe and North America. This figure has been redrawn from the original source [6] , but using lake-water DIN instead of DIN deposition, and adding data from the survey performed in the Pyrenees in 2000 (diamond, n =85). The solid line is the segmented regression fit used to establish the optimum breakpoint (vertical dashed line) between the DIN-dependent and DIN-independent segments, calculated using SegReg software [30] . Full size image The effects observed in the Pyrenees are likely occurring in other lake districts [15] , [16] . Here we present direct evidence, which was missing in previous studies, of the link between atmospheric P deposition and the N:P stoichiometry and the nutrient limitation status of phytoplankton in a lake. This provides a plausible explanation for the observed regional pattern of decreasing DIN in the whole Pyrenean lake district, and proves that increasing DIN deposition alone does not necessarily lead to increased DIN in lakes (and to a subsequent shift to phytoplankton P limitation) but that P deposition has also a role. This process is comparable to the atmospheric fertilization of remote areas of the open ocean, and may be included in the list of the biogeochemical effects of the global aerosol [17] . In our case, variations in the P load were attributed to changes in the natural fluxes driven by meteorology. Mineral aerosols are the main source of atmospheric P; however, human influence is already noticeable in the global atmospheric P cycle [8] and may eventually gain ecological relevance. Sampling Atmospheric bulk deposition, that is, wet (rain and snow) plus dry deposition, was sampled at the Centre for High Mountain Research station (CRAM, 42°37′16″N–0°45′58″E, 1,600 m asl) from 1997 to 2004, and at the Lake Redon station (formerly Lake Redó, 42°38′18″N–0°46′43″E, 2,240 m asl) during 1997–1998, 2000–2001 and from 2004 to the present. Despite the difference in altitude, these two stations are only ~2 km apart ( Supplementary Fig. S4 ). Samples from CRAM were collected on a daily basis in 1997 and 1998, and on a daily event basis thereafter. At the Lake Redon station, samples were collected monthly. The data series used in this study was constructed using information from the station that was in service in each given year, except for the water years 1997–1998 and 2000–2001 when both stations were run simultaneously. For these 2 years, the average was used, and the range of measurements is shown as error bars in the corresponding graphs. The agreement for these 2 years was good, thus allowing us to merge data to complete the series. Lake-water chemistry data come from Lake Redon [18] , [19] (24 ha, 73 m maximum depth, 32 m mean depth), and are volume-weighted averages from five sampling depths (2, 10, 20, 35 and 60 m) corresponding to the surface layer, epilimnion, metalimnion, upper (photic) hypolimnion and lower (dark) hypolimnion when the lake is stratified. The lake was monitored every fourth week, with a gap during 2002–2004 (due to financial problems). Stream chemistry was measured in the Conangles creek, close to CRAM ( Supplementary Fig. S4 ). The sampling point was at the outlet from the Conangles valley, an alpine watershed (7.6 km 2 , mean altitude 2,206 m asl, max altitude 2,887 m asl) located on a granodiorite bedrock, with a soil coverage of 77% (mainly alpine meadows and some pine forest in the lowest areas) and the remaining 33% scree and bare rock. The stream was sampled weekly from 1997 until 2001, and fortnightly thereafter. Synoptic sampling surveys covering the whole central Pyrenean lake district ( Supplementary Fig. S5 ) were conducted during the summer in 1987 (ref. 20 ), 1994–1996 (most lakes sampled in 1995), 2000 (ref. 21 ) and 2011. Chemistry was determined for the outflow water from the lakes, sampling either the surface layer or the outlet. The distribution of the major physiographic features of the surveyed lakes matched that of the inventory of the whole population: the lakes are distributed at altitudes between 1,620 and 2,990 m asl (average=2,300 m asl), their maximum depths are 0.7–123 m (average=16.5 m), their surface area ranges between 0.2 and 53.2 ha (average=5.5 ha) and the catchment area is 7–5,438 ha (average=115 ha). Their trophic status (year 2000 data) ranges between ultraoligotrophic to mesotrophic, with TP between 0.9 and 33 μg l −1 (average=5 μg l −1 ) and Chla (at the summer deep chlorophyll maximum) between <0.1 and 33 μg l −1 (average=2.1 μg l −1 ). Typical landcover in Pyrenean alpine catchments mainly consists of bare rock, scree and alpine meadows, with an average soil coverage of 40%. In the central Pyrenees, the predominant basin bedrock is granodiorite, with the presence of limestone and metamorphic rock (schist and slate) in some areas. Chemical analyses DIN was calculated as the sum of NO 3 − and NH 4 + . NO 3 − was measured by UV spectrophotometry [22] in the 1987 lake survey and by capillary electrophoresis (Quanta 4000, Waters) in all the remaining cases (lake, stream and atmospheric precipitation). NH 4 + in precipitation was measured by capillary electrophoresis; in stream and lake water, NH 4 + was measured by the classic blue indophenol method [23] . TP was analysed by the persulphate oxidation method [23] . Subsamples were first concentrated by evaporation with subsequent redissolution and oxidation of the residue with an acid potassium persulphate solution (20 ml evaporated sample to 2 ml final persulphate digest) followed by malachite green spectrophotometric determination of orthophosphate [24] in the digests. Chla in the lakes was determined by HPLC (Waters) in 90% acetone extracts of phytoplankton from the deep chlorophyll maximum collected on glass-fiber filters [25] . Data related to meteorology The duration of the ice cover and thermal stratification in Lake Redon was estimated using a thermistor (Vemco Minilog-TR) chain deployed at the deepest point of the lake. The first ice-free day was defined as the first day on which daily fluctuations caused by radiative heating were detected in the most surficial (2 m) thermistor. The last ice-free day was defined as the first day after the fall turnover on which the temperature at 2 m was consistently lower than at lower depths, thereby indicating the onset of inverse stratification. The first day of summer thermal stratification was defined as the first day after spring turnover on which temperature at 8 m differed from that at lower depths, thus indicating the formation of a well-established early seasonal thermocline. The last day of the summer stratification was defined as the first day on which temperature was homogeneous at all depths. The NAO index values used here were provided by the Historical Archive of Indices of the National Oceanic and Atmospheric Administration (NOAA) Climate Prediction Center [26] . Precipitation data were obtained from the automatic weather station (equipped with a Geonor T-200 snow/rain sensor and Campbell CR1000 data-logger) located at the sampling station at Lake Redon. How to cite this article: Camarero, L. & Catalan, J. Atmospheric phosphorus deposition may cause lakes to revert from phosphorus limitation back to nitrogen limitation. Nat. Commun. 3:1118 doi: 10.1038/ncomms2125 (2012).